Electric control of magnetism at the Fe/BaTiO3interface Interfacial magnetoelectric coupling is a viable path to achieve electrical writing of magnetic information in spintronic devices. For the prototypical Fe/BaTiO 3 system, only tiny changes of the interfacial Fe magnetic moment upon reversal of the BaTiO 3 dielectric polarization have been predicted so far. Here, by using X-ray magnetic circular dichroism in combination with high-resolution electron microscopy and first principles calculations, we report on an undisclosed physical mechanism for interfacial magnetoelectric coupling in the Fe/BaTiO 3 system. At this interface, an ultrathin oxidized iron layer exists, whose magnetization can be electrically and reversibly switched on and off at room temperature by reversing the BaTiO 3 polarization. The suppression/recovery of interfacial ferromagnetism results from the asymmetric effect that ionic displacements in BaTiO 3 produces on the exchange coupling constants in the interfacial-oxidized Fe layer. The observed giant magnetoelectric response holds potential for optimizing interfacial magnetoelectric coupling in view of efficient, low-power spintronic devices. The coupling of magnetization ( M ) and polarization ( P ) in multiferroic materials could permit to build up a new generation of memory devices, as it would exploit the best aspects of ferroelectricity (low-cost electric writing) and magnetism (robustness and durability of the stored information). In spite of recent progress in spin torque [1] , electric-field-assisted switching [2] or coherent magnetization switching [3] , magnetoelectric coupling (MEC) represents an advantageous route towards low-power electrical control, especially if reversible electric writing of the magnetic information, without need of auxiliary magnetic fields, could be achieved. Single-phase multiferroics [4] , [5] , [6] , [7] often present low Curie temperatures and weak MEC, thus hampering or limiting practical applications. Aiming at a large technological impact, multiferroic heterostructures, made of joint conventional ferromagnets (FMs) and traditional ferroelectrics (FEs), seem much more promising [8] , [9] . For the paradigmatic Fe/BaTiO 3 (BTO) system, sizable changes of the interfacial Fe magnetic moment upon reversal of the dielectric polarization of BTO have been predicted [10] , and huge variations of magnetoresistance have been observed by reversing the BTO polarization in Fe/BTO/La 2/3 Sr 1/3 MnO 3 (LSMO) tunnelling junctions [11] . Different mechanisms are currently explored in order to achieve electric-field control of MEC: (i) strain-mediated coupling at FM/piezoelectric interfaces [12] , [13] , [14] , (ii) exchange-bias coupling at FM/FE interface [15] , [16] , [17] , [18] , (iii) modulation of carrier density in the FM layer [19] , [20] , [21] , (iv) bond reconfiguration driven by ionic displacement at FM/FE interfaces [10] and (v) spin-dependent screening at FM/FE interfaces [22] . In this contribution, we report on a novel physical mechanism for MEC at the Fe/BTO interface. It has been proposed that interface cation displacements in BTO could give rise to a tiny variation of the Fe interfacial magnetic moment ( ∼ 10%), both for sharp [10] and oxidized interfaces [23] . Here we demonstrate, by X-ray magnetic circular dichroism (XMCD), that the magnetization of the interface spin system corresponding to the oxidized interfacial Fe layer (FeOx) can be reversibly switched on and off, at room temperature, by application of voltage pulses compatible with complementary metal-oxide semiconductor (CMOS) technology. First principles calculations, based on density functional theory, complemented by Hubbard-like corrections within the so called Density Functional Theory+U (DFT+U) approach, have been used to show that indeed, for reasonable U values, the exchange coupling constants in the adjacent FeOx layer can be largely reduced and even change sign by reversing the polarization of neighbouring BTO. Depending on the value of U used in calculations, this can simply lead to the weakening of FM ordering (and consequent decrease of the Curie temperature well below room temperature) or even to a transition from the FM to an anti-FM (AF) ground state, for large enough U values. In both cases, this scenario fully accounts for the observed room temperature switching of FM order in the FeOx layer. Noteworthy, we are dealing with an electrically induced change of the interfacial magnetic order, not simply with a reduction of the magnetic moment in a ferromagnetically coupled layer. The influence of an electric field ( E ) on the surface magnetization ( M s ) is usually described in terms of the surface magnetoelectric coefficient ( α s ) according to the following equation: μ o ΔM S = α s E . In our case, α s =2 × 10 −9 G cm 2 V −1 , corresponding to the complete switching of the interfacial layer magnetization. The observed ‘giant’ interfacial MEC thus largely exceeds predictions based on bond reconfiguration [10] or charge-screening mechanisms [22] . Samples growth In order to probe MEC at the Fe/BTO interface by XMCD, we fabricated some capacitors on epitaxial Au(4)/Co(1)/Fe(2 ML)/BTO(150)/LSMO(50)//SrTiO 3 (001) (Au/Co/Fe/BTO) heterostructures grown in situ (thicknesses in nanometres unless otherwise specified; ML, monolayer), where the limited thickness of the Fe layer allows XMCD probing the Fe interfacial properties and Co is introduced to stabilize ferromagnetism at room temperature (see below). Au(4)/Fe(1)/BTO(150)/LSMO(50)//SrTiO 3 (001) (Au/Fe/BTO) heterostructures, with a thicker Fe layer (1 nm), have been instead used to better investigate the interfacial Fe properties and their evolution towards the bulk properties in a continuous layer, less affected by the characteristic early-stage island growth of Fe on oxides. Transmission electron microscope investigation Electron microscopy observations denote high quality in our samples ( Fig. 1a,b ). A high-angle annular dark-field image obtained in an aberration-corrected scanning transmission electron microscope (STEM), on a [100] oriented slice from a Au/Fe/BTO sample, is shown in Fig. 1a . Brighter spots in the BTO region represent Ba–O columns and indicate that the BTO film is TiO 2 terminated. This can also be appreciated in the chemical colour maps in Fig. 1b , obtained from the electron energy-loss spectroscopy (EELS) analysis of the same interface. The enhanced red signal at the interface in Fig. 1b confirms the prevalence of the TiO 2 termination. The interfacial chemical sharpness can be better appreciated looking at the chemical profiles presented in Fig. 1c , which shows the normalized integrated intensities corresponding to the O–K (cyan), Ti–L 2,3 (red), Fe–L 2,3 (blue) and Ba–M 4,5 (green) edges. Apart from the evident TiO 2 termination, the signals from Ti and Fe decrease from 75 to 25% of the bulk value within a BTO unit cell, sign of an atomically sharp interface. Interestingly, we detect a significant amount of O beyond the BTO, into the interfacial Fe atomic plane, suggesting some degree of Fe oxidation at the interface plane. Unfortunately, the presence of beam broadening and dechanneling prevent us from being able of accurately determining the stoichiometry of the FeOx interfacial layer. However, its fingerprints are also present in the fine structure. In the right panel of Fig. 1a , we show the intensity ratio between the L 2 and L 3 components obtained from Fe–L 2,3 EEL spectra collected when scanning the sample along d , the growth direction marked with a cyan arrow. It can be appreciated that the L 23 intensity ratio is ∼ 3.7 away from the interface but it increases up to ∼ 4.2 at the interface. The L 23 ratio being a measure of the oxidation state of Fe ions, its enhancement signals the formation of an oxide layer confined at the Fe/TiO 2 interface, as reported earlier [24] . Further confirmation of the fact that the increase of L 23 ratio at surface indicates oxidation comes from the analysis of the O–K edge presented in Fig. 1d . In fact, the fine structure of the O–K edge depends directly on the bonding to the first neighbour cations. The red curve corresponds to the spectrum from the interface, whereas the black curve has been recorded within the BTO layer. The features corresponding to the perovskite-like fine structure of the black spectrum are smeared on the interface layer, and the appearance of the characteristic peak at ∼ 540 eV in the O–K spectrum from the interfacial Fe layer is consistent with the formation of a Fe oxide [25] . On the other hand, we can rule out the possibility that the increase of the L 23 ratio at the interface is due to screening of BTO surface charges, because the BTO slice used for TEM was un-poled, that is, broken in FE domains. As a matter of fact, we did measure the very same trend along the slice, without seeing any trace of inversion in the slope close to the interface, as expected in case of screening in proximity to domains with opposite polarization. 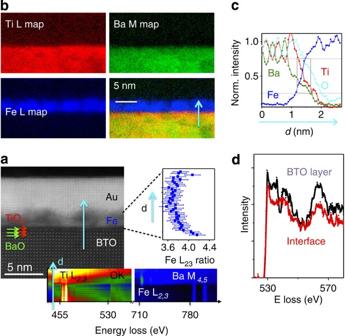Figure 1: TEM on Au/Fe/BaTiO3samples. Electron microscopy analysis of the Au(4)/Fe(1)/BTO(150)/LSMO(50)//SrTiO3(001) heterostructure (thicknesses in nanometres) used to study the interfacial Fe properties. (a) The atomic resolution Z-contrast image shows the BTO/Fe/Au stacking, with BTO[001]//Fe[001] and Fe[110]//BTO[100]. The BaO (TiO2) atomic planes near the BTO/Fe interface are marked with green (red) arrows. The EELS linescan acquired along the direction of the blue arrow, including the Ti–L2,3, O–K, Fe-L2,3and Ba–M4,5edges across the heterostructure, are shown in the bottom inset. The corresponding Fe–L23intensity ratio across the Fe layer (obtained through the second derivative method) are shown in the right panel. Principal component analysis has been used to remove random noise from the linesman. (b) Elemental maps for the BTO/Fe/Au stacking: Fe-L2,3(blue), Ti–L2,3(red) and Ba–M4,5(green). The maps were obtained by integrating a 30-eV wide window under the respective edges of interest after background subtraction using a power law. The RGB overlay of the three maps is also shown (R=Ti, G=Ba, B=Fe). (c) Normalized (Norm.), elemental profiles obtained from an EELS linescan across the BTO/Fe interface (same colour code as inb). The interface is TiO2terminated. The signal from the Ti and Fe planes, facing each other, goes down from 75 to 25% of the bulk value within a unit cell (marked with a grey rectangle), when moving across the interface, thus indicating an atomically sharp interface. (d) O–K edge from EELS spectra taken in the BTO bulk (black line) and in the interfacial Fe plane (red). Figure 1: TEM on Au/Fe/BaTiO 3 samples. Electron microscopy analysis of the Au(4)/Fe(1)/BTO(150)/LSMO(50)//SrTiO 3 (001) heterostructure (thicknesses in nanometres) used to study the interfacial Fe properties. ( a ) The atomic resolution Z-contrast image shows the BTO/Fe/Au stacking, with BTO[001]//Fe[001] and Fe[110]//BTO[100]. The BaO (TiO 2 ) atomic planes near the BTO/Fe interface are marked with green (red) arrows. The EELS linescan acquired along the direction of the blue arrow, including the Ti–L 2,3 , O–K, Fe-L 2,3 and Ba–M 4,5 edges across the heterostructure, are shown in the bottom inset. The corresponding Fe–L 23 intensity ratio across the Fe layer (obtained through the second derivative method) are shown in the right panel. Principal component analysis has been used to remove random noise from the linesman. ( b ) Elemental maps for the BTO/Fe/Au stacking: Fe-L 2,3 (blue), Ti–L 2,3 (red) and Ba–M 4,5 (green). The maps were obtained by integrating a 30-eV wide window under the respective edges of interest after background subtraction using a power law. The RGB overlay of the three maps is also shown (R=Ti, G=Ba, B=Fe). ( c ) Normalized (Norm. ), elemental profiles obtained from an EELS linescan across the BTO/Fe interface (same colour code as in b ). The interface is TiO 2 terminated. The signal from the Ti and Fe planes, facing each other, goes down from 75 to 25% of the bulk value within a unit cell (marked with a grey rectangle), when moving across the interface, thus indicating an atomically sharp interface. ( d ) O–K edge from EELS spectra taken in the BTO bulk (black line) and in the interfacial Fe plane (red). Full size image Noteworthy, Fig. 1a,b reveals that even a 1-nm-thick Fe layer grows on BTO in a three-dimensional mode. This is better seen in the EELS elemental maps of the sample used for XMCD experiments (Au/Co/Fe/BTO) shown in Fig. 2a , with nominal Fe thickness of 2 ML. The Fe film appears non-uniform, with local thickness ranging from 1 to 4 Fe ML. As TEM averages over the slice thickness, this is consistent with the characteristic tendency of metals to form nanoislands at the early stage of growth onto oxides [26] , [27] . This observation is of relevance, as these Fe nanoislands are expected to be superparamagnetic (see below) and justifies the use of a thin Co capping to stabilize the FM behaviour of thin Fe layers (2 ML) as required for subsequent XMCD experiments. Finally, note that despite the detailed chemical and structural characterization of the Fe/BTO interface has been performed on the sample with 1-nm-thick Fe (Au/Fe/BTO), because of the lower complexity of TEM analysis on this sample, the obtained results hold true also for the Co-capped Fe/BTO heterostructures. In Fig. 2b , we report the EEL spectrum taken from interfacial Fe atoms in these samples from which a Fe–L 23 intensity ratio of ∼ 4.3 can be estimated. This is fully consistent with the ratio found in the thick Fe sample just at the interface with BTO ( Fig. 1a ), and confirms that in case of just 2 Fe ML samples, Fe atoms strongly interact with BTO and present a clear signature of oxidation. 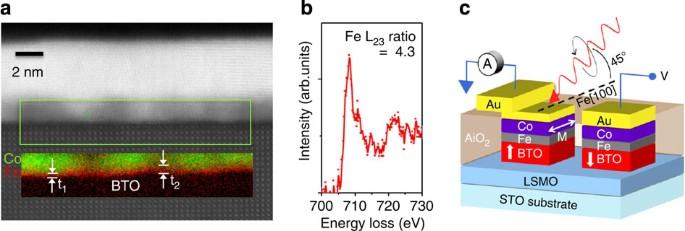Figure 2: TEM on Au/Co/Fe/BaTiO3samples and experiment layout. (a) STEM high-angle annular dark-field image (atomic resolution Z-contrast) and chemical colour map in a red-green overlay, (Co–L2,3map in green and the Fe–L2,3map in red) from the area marked with a green rectangle, acquired on the actual stack used for experiments: Co(1 nm)/Fe(2 ML)/BTO. The island growth mode of the Fe layer on BTO reflects in different thickness for the Fe layer, from∼1 ML (t1) to∼3–4 ML (t2). (b) Electron energy-loss spectrum taken from interfacial Fe atoms; arb., arbitrary. (c) Layout of the capacitors used for FE characterization and XMCD measurements under electric-bias condition. Figure 2: TEM on Au/Co/Fe/BaTiO 3 samples and experiment layout. ( a ) STEM high-angle annular dark-field image (atomic resolution Z-contrast) and chemical colour map in a red-green overlay, (Co–L 2,3 map in green and the Fe–L 2,3 map in red) from the area marked with a green rectangle, acquired on the actual stack used for experiments: Co(1 nm)/Fe(2 ML)/BTO. The island growth mode of the Fe layer on BTO reflects in different thickness for the Fe layer, from ∼ 1 ML (t 1 ) to ∼ 3–4 ML (t 2 ). ( b ) Electron energy-loss spectrum taken from interfacial Fe atoms; arb., arbitrary. ( c ) Layout of the capacitors used for FE characterization and XMCD measurements under electric-bias condition. Full size image FE characterization Capacitors were fabricated on Au/Co/Fe/BTO samples, according to a layout suitable for top-top FE measurements and XMCD under electric-bias condition ( Fig. 2c ). In the top-top configuration, two BTO capacitors are connected in series through the conducting LSMO electrode. Current ( I–E ) and polarization ( P–E ) loops of the very same capacitors used for subsequent XMCD experiments were measured at room temperature and 80 K. In Fig. 3a , we show the dynamic I–E characteristics measured at room temperature and at 100 Hz on Au(4)/Co(1)/Fe(2 ML)/BTO(150)/LSMO(50)//SrTiO 3 (001) capacitors with A 1 =0.02 mm 2 area. In the figure, the two current peaks associated to the switching of polarization are clearly seen, thus allowing the determination of the coercive field ( ∼ 120 kV cm −1 ). The P–E loop ( Fig. 3b ) indicates remanence and saturation polarization, P r =15 μC cm −2 and P s =30 μC cm −2 , which are characteristic of a good quality BTO. In Fig. 3c,d we show instead FE dynamic loops measured at 80 K on a different Au(4)/Co(1)/Fe(2 ML)/BTO(150)/LSMO(50)//SrTiO 3 sample, with capacitors area A 2 =1 mm 2 . Note that the coercive field is higher at low temperature ( ∼ 400 kV cm −1 ), as it can be inferred from Fig. 3c,d . From the dynamic P–E loop of Fig. 3d , P s =15 μC cm −2 and P r =10 μC cm −2 values can be extracted. 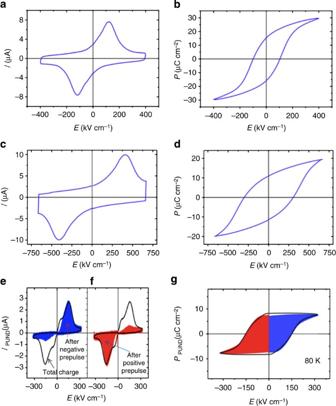Figure 3: FE characterization. (a)I–Echaracteristics recorded at room temperature and 100 Hz. (b)P–Edynamic loop obtained by integration through time of data ofa. (c)I–Echaracteristics and (d)P–Edynamic loop measured at 5 Hz and at 80 K. (e) The black line corresponds to a ‘standard’ PUND measurement. The blue line corresponds to PU and ND measurements after pre-polarizing the sample with −5 V pulse of 1 s and waiting 100 s. The blue dashed area for positiveEis proportional to the remanent charge 100 s after negative poling. (f) Black line idem toe, whereas the red line corresponds to PU and ND measurements after pre-polarizing the sample with +5 V pulse of 1 s and waiting 100 s. (g) Black line: polarization versus voltage loop obtained from the integration through time of the current measured in a complete PUND measurement. The blue (red) line and area correspond to the portion of the polarization loop obtained by integration of the PU (ND) measurement performed 100 s after pre-polarizing the sample with −5 V (+5 V). The strong similarity between the black loop and the blue-red one indicates good polarization retention after 100 s. Figure 3: FE characterization. ( a ) I–E characteristics recorded at room temperature and 100 Hz. ( b ) P–E dynamic loop obtained by integration through time of data of a . ( c ) I–E characteristics and ( d ) P–E dynamic loop measured at 5 Hz and at 80 K. ( e ) The black line corresponds to a ‘standard’ PUND measurement. The blue line corresponds to PU and ND measurements after pre-polarizing the sample with −5 V pulse of 1 s and waiting 100 s. The blue dashed area for positive E is proportional to the remanent charge 100 s after negative poling. ( f ) Black line idem to e , whereas the red line corresponds to PU and ND measurements after pre-polarizing the sample with +5 V pulse of 1 s and waiting 100 s. ( g ) Black line: polarization versus voltage loop obtained from the integration through time of the current measured in a complete PUND measurement. The blue (red) line and area correspond to the portion of the polarization loop obtained by integration of the PU (ND) measurement performed 100 s after pre-polarizing the sample with −5 V (+5 V). The strong similarity between the black loop and the blue-red one indicates good polarization retention after 100 s. Full size image We have assessed the retention of BTO at room temperature, under specific conditions, mimicking the protocol to be followed in the XMCD experiments. After application of pre-polarization pulses of 170 kV cm −1 (5 V) during 1 s, we waited for 100 s (that is, the characteristic time required for a single sweep of the Fe–L 2,3 XMCD spectrum) and then determined the final FE polar state with distinct positive-up (PU) and negative-down (ND) reading measurements at 340 kV cm −1 and delay time of 1 ms between P and U (N and D) [28] . In Fig. 3e,f in black is displayed the ‘standard’ PUND measurement [29] , without pre-polarization and 100 s waiting time, after appropriate subtraction of U from P and D from N. Therefore, the area under the black line in Fig. 3e is proportional to the total switchable polarization. The blue line, instead, corresponds to distinct reading PU and ND measurements, each of them performed after pre-polarizing the sample in the mentioned conditions with negative voltage. We can infer that the PU signal (positive voltages side) is almost equal to the measured PU signal in a complete PUND measurement. This denotes that almost 100% of the switchable charge has been switched by the pre-pulse and retained after 100 s. The opposite occurs for the ND signal (negative side), where the switchable current is almost zero. When the pre-polarizing voltage is positive (red line in Fig. 3f ), the situation is the same than that shown in Fig. 3e but with the opposite sign. Note that the sum of PU- and ND-dashed areas, proportional to the switchable charge, in both measurements is >100%. This is because the pre-polarizing 170 kV cm −1 pulse has not completely saturated the sample, contrary to that done in ‘standard’ PUND measurements, by using 340 kV cm −1 pulses. The ‘static’ P–E loops obtained from PUND measurements are reported in Fig. 3g . The room temperature standard P–E loop (black line) indicates a coercive field E C =150 kV cm −1 and a remanence polarization of ∼ 10 μC cm −2 . These values are slightly different from those obtained from the dynamic loops because of the different regime probed at 100 Hz and in the ‘static’ condition of PUND. In the same figure, the loop ‘in remanence’, made of blue and red lines, corresponds to distinct PU and ND measurements performed 100 s after pre-polarization. The fact that the two loops are almost identical indicates that, 100 s after application of the pre-polarization pulse, the remanent switchable charge is still 10 μC cm −2 , whereas sizable depolarization takes place over much longer times. XAS and XMCD X-ray absorption spectroscopy (XAS) and XMCD experiments have been performed both at room temperature and at 80 K. XAS spectra of the L 2,3 edge of Fe and Co have been collected in total electron yield, for a fixed light helicity (σ + and σ − ) and magnetization direction (m + and m − ) as sketched in Fig. 2c . A single-photon energy sweep took ∼ 100 s, which is compatible with an almost full retention of polarization (see above). A decrease of the XMCD signals from the interfacial-oxidized layer has been observed only over longer times, on the order of tens of minutes ( Supplementary Fig. 1 and Supplementary Note 1 ), so that our procedure of poling the sample before each scan ensures that experiments are performed at almost constant dielectric polarization of BTO. Let us first discuss the shape of XAS spectra and the influence of the Co overlayer on the magnetic properties of the 2-ML-thick Fe film in contact with BTO. In Fig. 4a,b , we show Co-L 2,3 and Fe–L 2,3 absorption spectra, respectively, taken at room temperature on Au/Co/Fe/BTO capacitors with 1-nm-thick Co layer and 2 ML of Fe. In Fig. 4b spectra-labelled S1 (S2) correspond to the addition of Fe–L 2,3 spectra collected with (σ + , m + ) and (σ − , m − ) ((σ + , m − ) and (σ − , m + )). We will focus on the L 3 edge where the intensity is higher and background subtraction is less critical. The prominent L 3 edge is constituted by a main component at 707.4 eV, corresponding to metallic Fe 0 , and a shoulder appearing at higher energy ( ∼ 709 eV), indicating a distinguishable oxidized Fe m+ state [30] , [31] . XAS data fully confirm the EELS data of Figs 1 and 2 , indicating the existence of an interfacial-oxidized iron layer that corresponds to Fe atoms in chemical interaction with BTO. As the crystal field and atomic environment of Fe atoms in this oxidized layer, sandwiched between BTO and metallic iron, are completely different from any of the well-known bulk Fe oxides, throughout all the paper we simply refer to it as ‘oxidized iron’ layer (FeOx). In Fig. 4b , we notice a clear dichroic signal in correspondence of the L 3 Fe edge (difference between S1 and S2 spectra), thus indicating FM order in the ultrathin Fe layer capped with 1 nm of Co. In Fig. 4c,d , instead, we show Co–L 2,3 (Fe–L 2,3 ) spectra taken at room temperature on Au/Co/Fe/BTO capacitors with lower Co thickness ( ∼ 0.1 nm). We can notice in this case the presence of an important FeOx component at higher energy compared with Fe 0 peak, maybe because of the absence of the Co barrier against oxidation. Moreover, we cannot observe any dichroic signal corresponding to the Fe edge (S1=S2). This finding underlines the importance of the role of Co in stabilizing a non-oxidized and FM ultrathin Fe layer on BTO surface. Without Co, Fe islands corresponding to the nominal thickness of 2 ML behave as superparamagnetic particles, with no remanent net magnetization at room temperature. 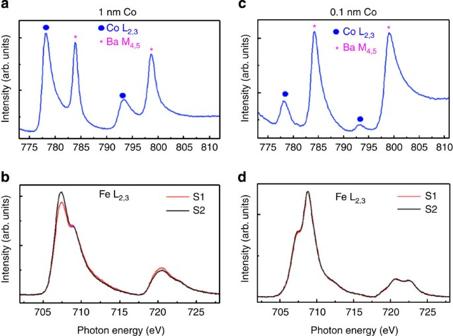Figure 4: XMCD after FE depolarization. (a) S1+S2 signal at Co–L2,3edge, (b) (S1 and S2 spectra collected at Fe–L2,3edge) taken at room temperature on Au/Co/Fe/BTO/LSMO//STO capacitors in case of 1-nm-thick Co layer. (c,d) As mentioned ina,bbut in case of a sample with 0.1 nm of Co. In this case, no evidence for ferromagnetism is found, thus indicating that a thick enough Co overlayer (1 nm) is needed to stabilize ferromagnetism within the two nominal MLs of Fe on BTO. Energy peaks indicated with stars in the top panels correspond to Ba–M4,5. Arb., arbitary. Figure 4: XMCD after FE depolarization. ( a ) S1+S2 signal at Co–L 2,3 edge, ( b ) (S1 and S2 spectra collected at Fe–L 2,3 edge) taken at room temperature on Au/Co/Fe/BTO/LSMO//STO capacitors in case of 1-nm-thick Co layer. ( c , d ) As mentioned in a , b but in case of a sample with 0.1 nm of Co. In this case, no evidence for ferromagnetism is found, thus indicating that a thick enough Co overlayer (1 nm) is needed to stabilize ferromagnetism within the two nominal MLs of Fe on BTO. Energy peaks indicated with stars in the top panels correspond to Ba–M 4,5 . Arb., arbitary. Full size image In Fig. 5a , we show the XAS Fe–L 2,3 spectra taken at room temperature on Au/Co/Fe/BTO capacitors after polarizing BTO with V + =+5 V ( E =170 kV cm −1 ) ( P up ). The difference of S1 and S2 spectra ( Fig. 5b ), normalized to the sum of their maximum at L 3 , is the XMCD that shows the expected prominent dichroic signal at the Fe 0 edge at 707.4 eV, but also a perceptible dichroism at the FeOx feature ( ∼ 709 eV). It is clear that both Fe 0 and FeOx edges contribute to the XMCD, thus signalling the presence of some net magnetization also in the FeOx layer, as indicated in the sketch in Fig. 5a (inset). In Fig. 5c , we show the corresponding XAS Fe–L 2,3 spectra taken on the same sample after polarization of BTO with V − =−5 V ( P dn ). Whereas S1 and S2 spectra largely differ at the Fe 0 edge, this difference disappears at the FeOx edge ( ∼ 709 eV, black arrow). This is better seen in Fig. 5b , where the XMCD data for P dn (red squares) are plotted. The comparison between XMCD for P up and P dn in Fig. 5b clearly shows that the dichroic signal of FeOx has been suppressed for P dn . It thus follows that whereas for P up the FeOx interface has a remanent magnetization, this is not the case for P dn that induces the transition of FeOx into either a non-magnetic or AF state as sketched in Fig. 5c (inset). Note that a null XMCD could be measured also on magnetic materials, if M were perpendicular to k . However, in the used experimental setup, k was set at 45° from the sample normal, and we do not expect M to be at 90° from k because of shape and magneto-crystalline anisotropy. The absence of XMCD for P dn is thus clearly related to a null average magnetization. This switching is fully reversible, as we repeatedly measured similar spectra by subsequently switching the BTO polarization. Furthermore, the differences of XMCD between P up and P dn become negligible when the samples are allowed to depolarize before XAS measurements ( Supplementary Note 1 ), thus confirming that the magnetic switching is related to the dielectric polarization. 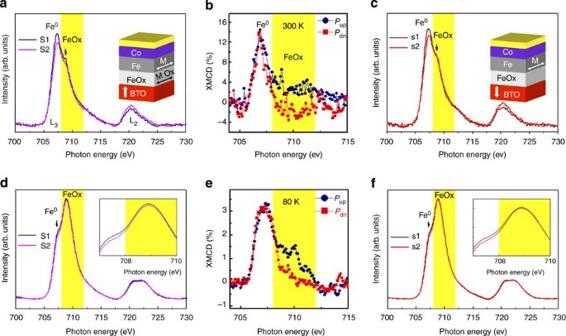Figure 5: XMCD for opposite BaTiO3FE polarization. (a,c) XAS Fe–L2,3spectra taken at room temperature on Au/Co/Fe(2 Ml)/BTO/LSMO//STO capacitors withA1=0.02 mm2area at 300 K after polarization of BTO withV+=+5 V (E=+170 kV cm−1) (Pup) andV−=−5 V (Pdn). (d,f) Experiments as mentioned in (a,b) but on capacitors withA2=1 mm2at 80 K. Insets in (a,c) are visual schemes of the Fe/BTO interface forPupandPdn: white vertical arrows correspond to BTO polarization direction, whereasMandMOxindicate the net magnetization in metallic Fe and in the FeOx layer at the Fe/BTO interface. Insets in (d,f) are zooms of the Fe–L3energy region. (b,e) XMCD signal in the Fe–L3energy region for BTO polarizationPup(blue circles) orPdn(red squares) taken on capacitors with area A1at 300 K and area A2at 80 K, respectively. The yellow shading indicates the region of the spectra corresponding to the oxidized Fe layer in contact with BTO. Figure 5: XMCD for opposite BaTiO 3 FE polarization. ( a , c ) XAS Fe–L 2,3 spectra taken at room temperature on Au/Co/Fe(2 Ml)/BTO/LSMO//STO capacitors with A 1 =0.02 mm 2 area at 300 K after polarization of BTO with V + =+5 V ( E =+170 kV cm −1 ) ( P up ) and V − =−5 V ( P dn ). ( d , f ) Experiments as mentioned in ( a , b ) but on capacitors with A 2 =1 mm 2 at 80 K. Insets in ( a , c ) are visual schemes of the Fe/BTO interface for P up and P dn : white vertical arrows correspond to BTO polarization direction, whereas M and MOx indicate the net magnetization in metallic Fe and in the FeOx layer at the Fe/BTO interface. Insets in ( d , f ) are zooms of the Fe–L 3 energy region. ( b , e ) XMCD signal in the Fe–L 3 energy region for BTO polarization P up (blue circles) or P dn (red squares) taken on capacitors with area A 1 at 300 K and area A 2 at 80 K, respectively. The yellow shading indicates the region of the spectra corresponding to the oxidized Fe layer in contact with BTO. Full size image In Fig. 5d,f , we show the XAS Fe–L 2,3 spectra taken at 80 K on a different Au/Co/Fe/BTO sample after polarizing BTO with V + ( P up ) and V − ( P dn ), respectively. In these large area capacitors, measurements at room temperature were prevented by the large leakage current in BTO. The FE coercive field is higher at 80 K than at room temperature (see above), but the application of ±5 V still results in a switching of BTO charges sizable enough to induce the magnetic switching. The relative weight of the Fe 0 and FeOx components differs compared with sample of Fig. 5a–c , most probably because of a slightly different actual coverage that results in a different degree of interfacial oxidation. However, of relevance here are the differences of XMCD obtained for P up and P dn as emphasized in Fig. 5e . In full agreement with data collected at room temperature shown in Fig. 5a–c , the dichroic signal of FeOx is largely suppressed for P dn . Being the XMCD proportional to the magnetization, data in Fig. 5a–f demonstrate that the magnetization of the interfacial FeOx can be electrically switched on and off by reversing the polarization of BTO. Whereas electro-induced Fe 0/m+ redox–oxidation process and concomitant changes of the relative weight of the FM (Fe 0 ) portion of the film at interfaces between metallic alloys and oxide surfaces have been reported [32] , we stress that in the present case magnetization switching occurs at FeO x layer without noticeable change of the oxidation state within the Fe film, as the average XAS lineshape is unchanged upon polarization reversal. We are facing a completely new mechanism for MEC, where the magnetic ordering of just interfacial Fe atoms is deeply affected, whereas ‘bulk’ metallic Fe atoms preserve their FM behaviour. This is in analogy with other recent findings on peculiar interfacial magnetic properties at Fe/oxides interfaces [33] . Density functional calculations To shed light on this marked magnetic reordering, we performed first principles density functional calculations. We simulated a supercell built by aligning the [100] axis of the TiO 2 -terminated BTO and the [110] axis of bct cobalt sandwiching (i) a single interfacial FeO layer and (ii) 1 FeO ML in contact with BTO, covered by 1 ML of ‘metallic’ Fe in contact with Co. Owing to the higher complexity of the analysis of exchange coupling constants in case (ii) and to the fact that case (i) is not unrealistic in our system (indeed Fig. 2a shows some portions of the film with ∼ 1 ML of oxidized Fe), we mainly present here results obtained for a single monolayer of FeO. The case (ii) of 2 Fe ML, corresponding to the nominal coverage used for the XMCD experiments, is presented in Supplementary Note 5 . However, we anticipate that the main results presented here for 1 ML hold true also for the 2 ML case. We used a Co (9 ML) overlayer and the thickness of BTO (8.5 ML) was chosen to ensure a bulk-like P in the middle of the layer. In Fig. 6a , we show the reconstructed Co/FeO/TiO 2 interfaces for P up (interface I) and P dn (interface II). For comparison, we also performed calculations for a ‘non-oxidized’ Fe layer, that is, using a Co/Fe/BaTiO 3 supercell stacking (similar to Fe/BaTiO 3 interface considered by Duan et al. [10] ) aiming to consider the two limiting extreme cases: a ‘fully oxidized’ case (FeO layer) and a ‘fully metallic’ (or ‘non-oxidized’) case (Fe layer). 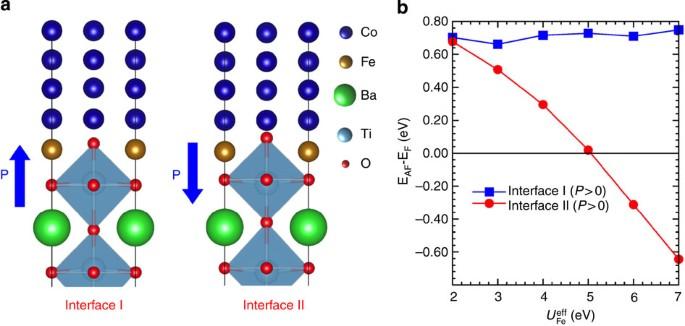Figure 6: DFT calculations. (a) Schematic plots of the simulated interface regions. From top to bottom: Co layer (blue spheres), FeO layer (light brown and red spheres for Fe and O, respectively) and BaTiO3layer (green, light blue and red spheres denote Ba, Ti and O, respectively). The left (right) panel shows interface I (II), in which the polarizationPup(Pdn) is pointing away from (towards) the BaTiO3layer, respectively. (b) Total energy changes (in eV and per unit cell) for FM and AF spin configurations of the interface Fe atoms, as a function of the HubbardUparameter within the DFT+U approach. Spin flips are carried out at interfaces I and II (see blue squares and red circles, respectively). Figure 6: DFT calculations. ( a ) Schematic plots of the simulated interface regions. From top to bottom: Co layer (blue spheres), FeO layer (light brown and red spheres for Fe and O, respectively) and BaTiO 3 layer (green, light blue and red spheres denote Ba, Ti and O, respectively). The left (right) panel shows interface I (II), in which the polarization P up ( P dn ) is pointing away from (towards) the BaTiO 3 layer, respectively. ( b ) Total energy changes (in eV and per unit cell) for FM and AF spin configurations of the interface Fe atoms, as a function of the Hubbard U parameter within the DFT+U approach. Spin flips are carried out at interfaces I and II (see blue squares and red circles, respectively). Full size image The GGA (Generalized Gradient Approximation)+U scheme was adopted to describe the d -electrons in Fe and Co. As the optimal value of U is in generally unknown, we allowed U ≡ U Fe – J Fe in the FeO layer to change in a wide range ( U ε[2:7] eV), whereas we kept U Co – J Co fixed at 2 eV for Co metallic layers. In order to assess the stability of the FM state, in Fig. 6b we plot the energy difference of the FeO interface with FM and AF spin order, the latter corresponding to reversing the spin direction of one of the two non-equivalent Fe atoms at the interface ( Supplementary Fig. 3 ). Note that this configuration is only one of the possible AF states corresponding to the minimum complexity allowing to perform DFT calculation within our cell structure. As shown in Fig. 6b , at U ∼ 5 eV, the FeO interface corresponding to P dn turns to be AF, whereas the FeO interface for P up remains FM; this effect is enhanced by further increasing U . These results show the tendency of the system towards a change in the magnetic order according to the sign of the BTO polarization. For the metallic Fe layer in the Co/Fe/BaTiO 3 heterostructure, a strong FM exchange interaction stabilizes the FM order and precludes any switch to an AF ground state upon polarization inversion ( Supplementary Fig. 2 ; Supplementary Tables 1 and 2 ; Supplementary Note 2 ). For Co/FeO/BTO heterostructures, we estimated the exchange coupling constants J Fe–Fe for nearest neighbour Fe spins as function of U , by mapping our DFT total energies to a simplified Heisenberg model. Consistent with data in Fig. 6b , we found that J Fe–Fe ( U ) weakens and has a sign inversion from FM to AF at U ∼ 3 eV, becoming more AF upon increasing U ( Supplementary Fig. 2 ). The modulation of the magnetic properties of the FeO layer, namely the switch from FM to AF character when switching the polarization of BTO, results from the polarization-induced atomic-position shifts and subsequent modifications of the Fe–O bond topology when interfaced with the TiO 2 surface of BTO. As explained in detail in the Supplementary Note 3 , the major bond reconfiguration concerns the coupling between the two non-equivalent Fe atoms, which is indeed mediated by the oxygen atom (O II) in the underlying TiO 2 plane. The position of the latter is severely affected when switching polarization ( Supplementary Table 3 ), thus leading to a large increase in the Fe-O II-Fe angle (from 96.7 up to 112.3 degrees) at interface II ( P dn ) with respect to interface I ( P up ). Correspondingly, also the Fe-O II bond length suffers from a sizable reduction (from 2.67 to 2.40 Å). As superexchange Fe-O-Fe interactions are known to be extremely sensitive to bond angle and distances, it is quite reasonable to guess that one of the two interfaces can develop a different magnetic order, in agreement with total energy DFT calculations. The presence of the FM Co layer tends to favour a FM order of the neighbouring FeOx layer, thus explaining why the AF order is only achieved at relatively large U . Indeed, the transition towards antiferromagnetism at interface II in the exchange coupling J Fe–Fe occurs at smaller values of U with respect to the total energy ( U >3 eV; Supplementary Fig. 2 ). As for the local electronic structure, we do not observe sizable changes within the FeO layer upon polarization reversal. The Fe magnetic moments are always ∼ 3.5 Bohr magnetons, and only a slight increase of the exchange splitting in the PDOS of the flipped Fe atoms is seen in the AF configuration for interface II ( P dn ) ( Supplementary Fig. 4 ; Supplementary Table 5 ; Supplementary Note 4 ), in agreement with the total energy decrease stabilizing AF in this case. As anticipated above, simulations performed on 2 ML of Fe on BTO display the same trend, that is, the stabilization of the AF order at high U for interface II ( Supplementary Fig. 5 , Supplementary Note 5 ) accompanied by a major bond reconfiguration driven by polarization reversal ( Supplementary Table 4 ). This is a strong indication of the robustness of the DFT analysis as well as of the proposed mechanism for the switching of the magnetic order. Note that our results represent a step forward with respect to pioneering calculations performed by Fechner et al. [34] for an oxidized ultrathin Fe layer on BTO. Although in a rather different geometry (that is, without Co-capping layer) and in different interfacial atomic configurations, those calculations showed FM coupling in the absence of electronic correlations (that is, within a bare local-spin-density approximation). We here demonstrated that the inclusion of ‘beyond-local-spin-density approximation/GGA’ approaches (such as DFT+U) markedly affects the magnetic coupling, and it is therefore required to achieve an accurate description of magnetoelectricity at the Fe/BTO interface. The weakening of the FM interaction for interface II ( P dn ) is fully coherent with the disappearance of XMCD from the interfacial FeOx layer for P dn . Depending on the strength of correlation effects, we could expect a transition to AF coupling or simply a weakening of exchange constants leading to a lowering of the interfacial Curie temperature below the minimum temperature of our experiments (80 K). As for the value of the Hubbard parameter, in literature widely spread values (ranging from 4.0 eV (ref. 35 ) to 4.8 eV (ref. 36 ) to 6.8 eV (ref. 37 )) are available for bulk FeO. Indeed, the situation we have of a thin oxidized Fe layer is very far from bulk FeO, and the low dimensionality might possibly induce large electronic correlations. However, even in the case of the lowest reported Hubbard value for the FeO compound, that is, U =4.0 eV (ref. 33 ) our calculation indicates a small energy difference between the FM and AF state (reduced by ∼ 50% with respect to bare GGA results). Looking at the exchange constants J Fe–Fe reported in the Supplementary Fig. 2 for the case of just 1 ML of FeO, we note that already for U =4 eV J Fe–Fe becomes negative. This confirms that the general trend suggested by our calculations, that is, the weakening of FM interaction at interface II eventually leading to an AF ground state for large U values, is fully compatible with realistic values for the Hubbard parameter. A more detailed investigation of the magnetic ordering of the ‘off’ magnetic state, for instance by X-ray linear dichroism, would be needed in order to elucidate if the ‘non-magnetic’ state is either paramagnetic or AF, but this is definitely beyond the scope of this work. To summarize, we have demonstrated a novel physical mechanism for interfacial MEC leading to a room temperature electrical and reversible on/off switching of the interfacial Fe magnetization in the Fe/BTO heterostructure. DFT+U calculations have shown that the FeO/BTO interfaces are markedly asymmetric with respect to the polarization of BTO, whereas the interface with P dn can undergo a magnetic transition towards an AF (or paramagnetic) state, the P up interface remains robustly FM. At variance with previous works dealing with MEC driven by bond reconfiguration [10] , we propose here a completely new mechanism based on the induced change of magnetic order, not simply on the change of the interfacial magnetic moments. As the magnetization of the FM layers corresponds to ∼ 3.5 μ B per atom, switching on/off the magnetization at E C leads to a record value of the surface MEC α s =2 × 10 −9 G cm 2 V −1 . This value exceeds previous predictions of MEC at Fe interfaces based on bond reconfiguration [10] and the spin-dependent screening mechanism [21] by one and four orders of magnitude, respectively. Finally, let us estimate the energy consumption for the switching of the magnetic ordering via reversal of the polarization. For a device constituted by a FM electrode of 50 nm diameter and BTO thickness of 15 nm, the switching of the polarization at E C would require ∼ 0.7 × 10 −16 J. This is of the same order of magnitude of the energy consumption reported in the case of coherent magnetization switching via voltage pulses assisted by external magnetic fields [2] , [3] and 1/500 times lower than that required for writing information via spin-current injection [1] . This confirms the great potential of the peculiar mechanism for MEC here disclosed to achieve a reversible, fully electrical writing of the magnetic information in spintronic devices, such as magnetic tunneling junctions, where the surface magnetization has a major role. Sample fabrication BTO/LSMO bilayers were grown by pulsed laser deposition on (001) SrTiO 3 (STO) substrates using a quadrupled Q-Switched Nd:YAG laser ( λ =266 nm) with a fluence of 5.2 J cm −2 (for LSMO deposition process) or 2.2 J cm −2 (for BTO deposition process) and a repetition rate of 2 Hz. LSMO films (50 nm) were grown at a deposition temperature of 730 °C and an oxygen pressure of 0.22 Torr. The subsequent growth of 150-nm-thick BTO, performed at 640 °C and with an oxygen pressure of 0.02 Torr, was followed by 30 min annealing at 600 °C in a high oxygen pressure (760 Torr). After cooling down to room temperature, Au(4)/Co(1)/Fe(2 ML) and Au(4)/Fe(1) (from now on thickness in nanometres unless otherwise specified), multilayers were grown in situ (without breaking the vacuum) by molecular beam epitaxy in a cluster tool system equipped with both pulsed laser deposition and molecular beam epitaxy facilities [38] . The pressure during the deposition process was always in the 10 −10 Torr range. Upon Fe deposition, a 20-min post annealing at 200 °C was performed in order to improve the structural quality of Fe. The deposition rates for Fe, Co and Au were calibrated with a quartz microbalance. Preliminary studies of growth mechanisms and dielectric properties of BTO epitaxial films indicate the good quality of the FE film grown in these conditions [39] . In situ low-energy electron diffraction and X-ray photoemission spectroscopy were used to optimize the epitaxial growth of Fe on BTO, starting from our previous work on the epitaxial growth of Fe on BTO (ref. 40 ), in order to improve crystallinity and achieve a sharp chemical interface, with a monolayer of oxidized iron at the interface. Capacitors, with A 1 =0.02 mm 2 and A 2 =1 mm 2 areas, were fabricated using optical lithography and ion milling, according to a layout showed in Fig. 2c . A SiO 2 layer was deposited by sputtering to allow the fabrication of the final Au(200)/Ti(15) contacts electrically connecting the top of the capacitors but only partially covering them, in order to leave part of the stack free for XMCD. STEM-EELS characterization Samples for STEM-EELS were prepared by conventional methods: polishing and Ar ion milling. The samples were studied in a Nion UltraSTEM200 operated at 200 kV and equipped with a fifth order Nion aberration corrector and a Gatan Enfinium spectrometer, and also in a Nion UltraSTEM100 operated at 100 kV equipped with a Nion aberration corrector and a Gatan Enfina spectrometer. In some cases, random noise was removed by using principal component analysis. FE characterization A symmetric planar capacitor configuration with top contacts was used to record current versus electric field (TF Analyzer 2000 from AixACCT Co). From the integration of the recorded current versus time, normalized to the electrode area, the polarization ( P ) was obtained. Conventional P–E loops have been measured with the PUND technique, whereas loops ‘in remanence’, to explore polarization retention, were measured as follows. After application of pre-polarization pulses of 5 V during 1 s and a delay time of 100 s (that is, the characteristic conditions for a single sweep of the Fe–L 2,3 XMCD spectrum), we determined the final FE polar state with selective PU and ND reading measurements at 10 V (2.5 ms pulse duration with triangular shape) and delay time of 1 ms. This gives access to the total amount of switched charge by the pre-polarizing pulse. Additional experimental details on the FE measurements are reported elsewhere [26] , [27] . XMCD measurements XMCD experiments have been carried out at the APE beamline of the ELETTRA synchrotron radiation source. XAS spectra of the L 2,3 edge of Fe and Co have been collected in total electron yield with fast scan mode, that is, by changing the incoming photon energy in a continuous way while measuring the sample drain current by means of a picoammeter inserted between the surface of the sample and ground, for a fixed light helicity (σ + and σ − ) and magnetization direction (m + and m − ) as sketched in Fig. 2c . The polarization state of the sample has been fixed as follows. Before any photon energy scan, the BTO was poled with a positive or negative voltage pulse ( V =±5 V) applied to the LSMO bottom layer, thus setting a BTO polarization pointing towards ( P up ; V + ) or outwards ( P dn ; V − ) the Fe layer, respectively. For each FE polarization state ( P up , P dn ), XAS spectra have been collected for the different combinations of light helicity (σ +/− =±80%) and sample magnetization (m +/− , corresponding to saturation long the [100] and [−100] directions) in order to get rid of instrumental asymmetries. The angle of incidence of the incoming light was kept fixed at 45 degrees with respect to the direction of the magnetizing field, parallel to the Fe[100] easy axis in the sample surface, while the light azimuth was the Fe[100] direction. In the XAS measurement, data have been taken in magnetic remanence, upon application of magnetic pulses of 200 Oe. Spectra have been normalized in order to take into account the 45 degrees angle between the photon angular momentum and magnetization, as well as the non-unitary value of the light helicity. First principles calculations Density functional theory simulations were performed by using the Vienna Ab initio Simulation Package [41] . The ion-electron interaction was treated by means of the projector augmented wave pseudo-potentials. The exchange and correlation terms were considered within the GGA in the Perdew–Burke–Ernzerhof formalism [42] . We have used an energy cutoff for the plane wave basis as large as 500 eV, a Brillouin zone sampled over the 10 × 10 × 1 Monkhorst–Pack k-point mesh [43] , whereas the internal coordinates have been optimized until the forces on all atoms became <0.02 eV Å −1 . Finally, GGA+U calculations were performed following Dudarev's formulation [44] . The in-plane lattice constant has been fixed at the experimental value for BTO ( a = b =3.991 Å), whereas the out of plane one (c) has been chosen in a way so as to minimize the supercell total energy. How to cite this article : Radaelli, G. et al. Electric control of magnetism at the Fe/BaTiO 3 interface. Nat. Commun. 5:3404 doi: 10.1038/ncomms4404 (2014).